Room-temperature sub-band gap optoelectronic response of hyperdoped silicon Room-temperature infrared sub-band gap photoresponse in silicon is of interest for telecommunications, imaging and solid-state energy conversion. Attempts to induce infrared response in silicon largely centred on combining the modification of its electronic structure via controlled defect formation (for example, vacancies and dislocations) with waveguide coupling, or integration with foreign materials. Impurity-mediated sub-band gap photoresponse in silicon is an alternative to these methods but it has only been studied at low temperature. Here we demonstrate impurity-mediated room-temperature sub-band gap photoresponse in single-crystal silicon-based planar photodiodes. A rapid and repeatable laser-based hyperdoping method incorporates supersaturated gold dopant concentrations on the order of 10 20 cm −3 into a single-crystal surface layer ~150 nm thin. We demonstrate room-temperature silicon spectral response extending to wavelengths as long as 2,200 nm, with response increasing monotonically with supersaturated gold dopant concentration. This hyperdoping approach offers a possible path to tunable, broadband infrared imaging using silicon at room temperature. Developing a low-cost broadband infrared detector with array-based real-time imaging capability at room temperature is of interest for telecommunications, security, energy and research and development applications [1] , [2] , [4] , [5] . Silicon-based detectors satisfy the low-cost and on-chip complementary metal-oxide semiconductor (CMOS) compatibility criteria, but their infrared photoresponse is fundamentally limited by the 1.12-eV band gap ( λ =1,110 nm). Previous attempts to extend the photoresponse of silicon-based devices into the short-wavelength infrared regime ( λ =1,400–3,000 nm) at room temperature focused on forming heterostructures with SiGe alloys [6] , [7] , [8] or microstructures of thermally absorbing material [9] , [10] , and modifying the intrinsic band structure via intentional introduction of defects [11] , [12] , [13] , [14] , [15] , [16] , [17] . Growing microstructures of foreign materials on top of silicon results in processing complexities that can compromise CMOS compatibility [18] , [19] . Furthermore, integration of thermally absorbing materials can be effective for short-wavelength infrared response but results in slow pixel response times intrinsically limited by the thermal time constant, which hinders applications in array-based real-time imaging systems at room temperature [10] . The direct modification of silicon’s electronic band structure is a promising approach for imaging applications, but significant advances on room-temperature sub-band gap photoresponse in silicon to date are mostly focused on fiber-coupled single-point detector applications. Published approaches predominantly involve intentionally damaging the silicon lattice [12] , [13] , [14] , [15] , [16] , [17] , which produces a measurable sub-band gap absorption coefficient ( α =2–4 cm −1 ) [16] compared with untreated silicon ( α <2 × 10 −7 cm −1 for λ >1,400 nm) [20] . To increase the optical path length and sub-band gap absorptance, these devices are integrated with micron-sized waveguide resonators [13] , [17] . By intentionally damaging the silicon lattice, Geis et al . [16] fabricated single-point, fibre-coupled waveguide photodiodes and phototransistors with room-temperature sub-band gap ( λ =1,550 nm) photoresponse of 20 and 50 A W −1 , respectively [16] , [17] . These results correspond to impressive quantum efficiencies of 16 and 40, much larger than unity because of avalanche gain [16] , [17] . Unfortunately, the waveguide architecture renders this device responsive for only a narrow band of wavelengths, and the requirement for coplanar illumination impedes incorporation into imaging arrays. Another approach involves incorporating chalcogen dopants into silicon through picosecond or femtosecond laser irradiation. This approach has resulted in a limited number of reports of infrared photoresponse [21] , [22] . However, the origin of the sub-band gap photoresponse is not well understood or controlled owing to the complexity of the laser-processed microstructure involving structural defects and multiple chemical phases [23] . To elucidate the origin of sub-band gap photoresponse in chalcogen-doped silicon, sulphur ions have been implanted into silicon and the resulting amorphous layer subjected to pulsed laser melting (PLM)-induced rapid solidification using a nanosecond laser, resulting in a single-crystalline silicon layer with sulphur concentrations above 10 19 cm –3 (ref. 24 ). This nanosecond laser-hyperdoping process is repeatable and yields homogenous and single-crystal material, reducing the material’s complexity compared with the microstructure with multiple phases found in silicon irradiated with picosecond or femtosecond lasers [23] . However, there are no reports of room-temperature sub-band gap photoresponse for this single-crystalline material. As chalcogen hyperdoping introduces only donor states into the silicon band gap, the resulting material has a large background-free carrier concentration at room-temperature [25] , [26] . This large background-free carrier concentration overwhelms the sub-band gap photoconductivity signal, making the observation of room-temperature sub-band gap photoconductivity in chalgogen-hyperdoped silicon difficult [27] . Similar problems have been encountered in titanium-hyperdoped silicon for which sub-band gap photoconductivity is observed only at liquid nitrogen temperature or below [28] . This is similar to prior work on impurity-diffused silicon photodetectors where the demonstration of sub-band gap photoresponse has been limited to low temperatures [29] , [30] . Room-temperature sub-band gap photoresponse of hyperdoped single-crystalline silicon remains elusive. In this study, we report room-temperature sub-band gap photoresponse from single-crystalline silicon hyperdoped with an alternative dopant, gold, to concentrations as high as 5 × 10 20 cm –3 . We present planar photodiode devices suitable for imaging-array applications fabricated from silicon hyperdoped with gold (Si:Au). Steady-state and transient photoresponse measurements demonstrate that the photodiode optoelectronic response extends well into the sub-band gap regime of silicon, to at least λ =2,200 nm. Furthermore, the magnitude of the response increases monotonically with gold dopant concentration. The homogenous, single-crystalline nature of Si:Au gives insight into the likely physical mechanism of enhanced sub-band gap photoresponse, a discrete set of Au-induced donor and acceptor mid-gap energy levels that generate free carriers in response to infrared light, yet reduce background-free carrier concentrations via self-compensation. As PLM induces substantial heating only in the top 150 nm of the wafer, it might be added as the last step of any CMOS-compatible optoelectronic device fabrication process in user-defined device areas, limiting potential unintentional contamination effects of Au. Gold hyperdoping of silicon The top 150 nm of three identical <100> n -type silicon wafers were implanted with gold ions using an implantation energy of 50 keV and doses of 3 × 10 14 , 7 × 10 14 and 1 × 10 15 cm −2 . PLM was used to melt the amorphous implanted region, which rapidly solidifies back into single-crystal silicon with high, non-equilibrium dopant concentration ( Fig. 1a ) [24] . Because of gold’s high diffusive velocity and segregation coefficient in liquid silicon [31] , the high solidification speed outpaces the kinetics of gold segregation and results in a supersaturated, single-crystalline solid solution [31] , [32] . An Nd:YAG nanosecond pulse was used to melt and rapidly solidify the gold-hyperdoped silicon (Si:Au) region, and in situ time-resolved reflectivity [33] measurements showed a melt duration of 25–30 ns, corresponding to a solidification speed of about 7–10 m s −1 based on a dopant diffusion simulation in established literature [31] . This process is represented pictorially in Fig. 1a ; more detail about the PLM process can be found in the Methods section. 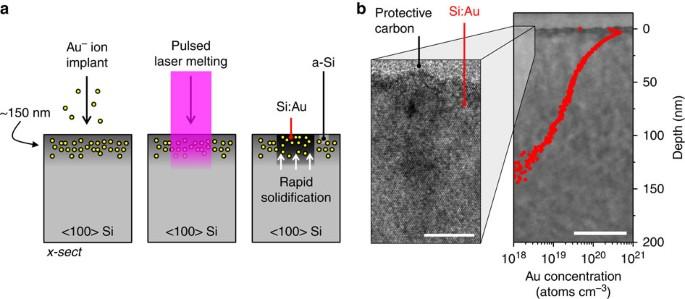Figure 1: Fabrication of Si:Au. (a) Fabrication of Si:Au: ion implantation of Au followed by PLM. Rapid solidification follows the PLM process, producing single-crystalline Si:Au on the top 150 nm of the silicon wafer. The silicon area not melted by the PLM remains amorphous. (b) SIMS profile of Si:Au with 1 × 1015cm−2gold implantation dose, showing that the gold concentration in the Si:Au is more than four orders of magnitudes beyond the solid solubility limit of gold in silicon. The transmission electron microscopic images show that for this gold implantation dose, the entire Si:Au layer is crystalline. Scale bar, 10 nm (left) and 50 nm (right). Figure 1: Fabrication of Si:Au. ( a ) Fabrication of Si:Au: ion implantation of Au followed by PLM. Rapid solidification follows the PLM process, producing single-crystalline Si:Au on the top 150 nm of the silicon wafer. The silicon area not melted by the PLM remains amorphous. ( b ) SIMS profile of Si:Au with 1 × 10 15 cm −2 gold implantation dose, showing that the gold concentration in the Si:Au is more than four orders of magnitudes beyond the solid solubility limit of gold in silicon. The transmission electron microscopic images show that for this gold implantation dose, the entire Si:Au layer is crystalline. Scale bar, 10 nm (left) and 50 nm (right). Full size image After PLM, secondary ion mass spectrometry (SIMS) was performed to measure the gold atomic concentration as a function of depth ( Fig. 1b ). The solid solubility limit of gold in silicon at room temperature is estimated to be below 10 15 cm −3 (refs 34 , 35 , 36 , 37 ). Supersaturated gold concentrations were achieved up to 150 nm depth for all three gold doses, with the largest gold concentration peak of 5 × 10 20 cm −3 measured within the top 10 nm of the Si:Au layer. This corresponds to 1 at.% Au concentration, more than four orders of magnitude above the room-temperature equilibrium solid solubility limit of gold in silicon. High-resolution transmission electron microscopic measurements confirmed that the entire Si:Au layer was single crystalline, without formation of any extended defects, secondary phases or cellular breakdown ( Fig. 1b ) [38] . Because of the large concentration of mid-gap dopant levels introduced by the gold impurities, the hyperdoped layer absorbs sub-band gap light as shown in the infrared transmission image through the sample taken using an InGaAs camera ( Fig. 2a ). Transmission ( T ) and reflection ( R ) were measured using ultraviolet–visible–near-infrared spectrophotometry to quantify the sub-band gap absorptance ( A = 1 − T − R ) in the hyperdoped silicon. Similar to chalcogen-hyperdoped silicon [39] , sub-band gap light absorptance increases with increasing Au concentration ( Fig. 2b ). Approximating the sub-band gap absorptance occurring uniformly throughout the hyperdoped region (150 nm thickness), the average sub-band gap absorption coefficient α at λ =1,550 nm of the Si:Au with the highest gold dose is estimated to be about 600 cm −1 (1% absorptance averaged over a 150-nm thick layer; see Methods ), which is larger than that of germanium at the same wavelength (~300 cm −1 ) [40] . 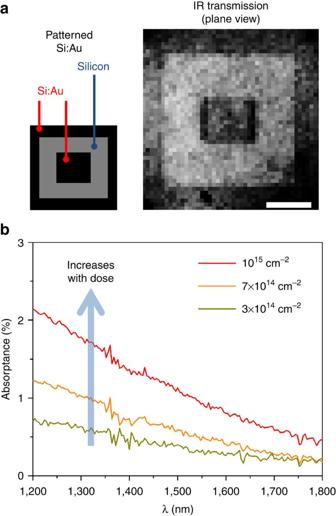Figure 2: Sub-band gap absorptance of Si:Au. (a) Transmission of sub-band gap light through patterned Si:Au taken using an InGaAs camera. Light transmission is reduced by absorption in Si:Au (dark areas) relative to the crystalline silicon (bright areas). Scale bar, 1 mm. (b) Sub-band gap light absorptance (1—transmission—reflection) of Si:Au for various gold implantation dose relative to the sub-band gap light absorptance in the reference plain silicon sample, measured using ultraviolet–visible–near-infrared spectrophotometry. Sub-band gap light absorptance increases with increasing gold dose. Figure 2: Sub-band gap absorptance of Si:Au. ( a ) Transmission of sub-band gap light through patterned Si:Au taken using an InGaAs camera. Light transmission is reduced by absorption in Si:Au (dark areas) relative to the crystalline silicon (bright areas). Scale bar, 1 mm. ( b ) Sub-band gap light absorptance (1—transmission—reflection) of Si:Au for various gold implantation dose relative to the sub-band gap light absorptance in the reference plain silicon sample, measured using ultraviolet–visible–near-infrared spectrophotometry. Sub-band gap light absorptance increases with increasing gold dose. Full size image Steady-state room-temperature sub-band gap photoresponse To measure the room-temperature sub-band gap photoresponse in Si:Au, photodiodes were fabricated (see Methods ). The dark I–V curves ( Fig. 3b ) for photodiodes fabricated on n -type silicon substrates exhibit rectification behaviour, as expected when the majority carriers in supersaturated Si:Au are holes [41] . In contrast, Si:Au on a p -type Si substrate does not show rectification ( Supplementary Fig. 1 ). Reactive ion etching and electron-beam Ti/Au contact evaporation were used to electrically isolate and contact a 1 × 1 mm 2 (ref. 2 ) Si:Au area to define the active area of the device. An identical photodiode was fabricated on the same substrate but with the Si:Au layer replaced by boron-doped silicon (Si:B) as a reference sample ( Supplementary Fig. 2 ). 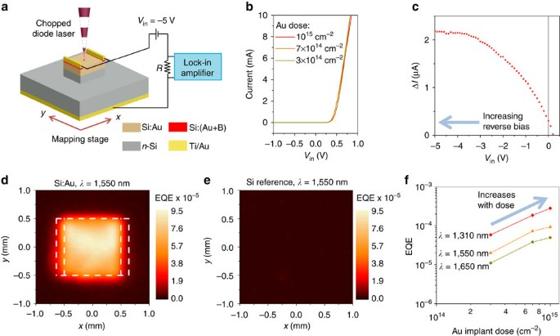Figure 3: Room-temperature sub-band gap photoresponse in Si:Au. (a) Si:Au photodiode with Si:Au layer onn-Si substrate operating at reverse bias. The optically chopped diode laser light is focused to 100–150 μm spot size and is scanned across the photodiode surface. (b) The darkI–Vcurve of Si:Au onn-type Si shows rectification behaviour for gold implantation dose of 3 × 1014–1 × 1015cm−2, indicating that the majority carriers in Si:Au are holes. (c) The difference between dark and illuminatedI–Vof the photodiode with 1015cm−2gold dose. Increasing reverse bias across the junction increased carrier drift velocity in the Si:Au layer, improving the collection of photo carriers excited by the sub-band gap light. (d) Mapped external quantum efficiency (EQE) showing a 1 × 1 mm2Si:Au active area forλ=1,550 nm and gold implantation dose of 1015cm−2, confirming the Si:Au layer as the sole source of the sub-band gap photoresponse in the photodiode. (e) No sub-band gap response is observed when the Si:Au is replaced with Si:B in the reference silicon photodiode. (f) EQE for various sub-band gap wavelengths increases with the gold concentration in the Si:Au photodiode. Figure 3: Room-temperature sub-band gap photoresponse in Si:Au. ( a ) Si:Au photodiode with Si:Au layer on n -Si substrate operating at reverse bias. The optically chopped diode laser light is focused to 100–150 μm spot size and is scanned across the photodiode surface. ( b ) The dark I–V curve of Si:Au on n -type Si shows rectification behaviour for gold implantation dose of 3 × 10 14 –1 × 10 15 cm −2 , indicating that the majority carriers in Si:Au are holes. ( c ) The difference between dark and illuminated I–V of the photodiode with 10 15 cm −2 gold dose. Increasing reverse bias across the junction increased carrier drift velocity in the Si:Au layer, improving the collection of photo carriers excited by the sub-band gap light. ( d ) Mapped external quantum efficiency (EQE) showing a 1 × 1 mm 2 Si:Au active area for λ =1,550 nm and gold implantation dose of 10 15 cm −2 , confirming the Si:Au layer as the sole source of the sub-band gap photoresponse in the photodiode. ( e ) No sub-band gap response is observed when the Si:Au is replaced with Si:B in the reference silicon photodiode. ( f ) EQE for various sub-band gap wavelengths increases with the gold concentration in the Si:Au photodiode. Full size image The photodiodes were then connected to a comparative resistor, a lock-in amplifier and a voltage source ( V IN =−5 V) that placed the devices under reverse bias ( Fig. 3a ). A diode laser (optically chopped at frequency f =714 Hz) was focused to a 100–150-μm spot size on the photodiode surface. The comparative resistor value of R =1 kΩ was chosen such that the reverse bias voltage across the photodiodes was close to 5 V ( I dark R <<| V in |). The laser spot was then scanned across the photodiode surface. Sub-band gap optoelectronic response was observed only in the 1 × 1-mm 2 area of the photodiode corresponding to the electrically connected Si:Au region. A map of sub-band gap response at λ =1,550 nm is shown in Fig. 3d for a sample with implantation dose of 10 15 Au cm −2 . The spatial uniformity of the photoresponse within the 1 × 1-mm 2 area demonstrates that internal photoemission from the metal contact electrodes is not the dominant cause of the sub-band gap photoresponse [42] . The reference Si:B photodiode control samples did not show any measurable sub-band gap optoelectronic response ( Fig. 3e ), further confirming that the Si:Au layer is the origin of the room-temperature sub-band gap photoresponse. This observation is in contrast with the low-temperature sub-band gap photoresponse previously reported in titanium-hyperdoped silicon, where the sub-band gap photoresponse of the reference crystalline silicon is reported to be larger than that of the titanium-hyperdoped silicon [43] . The sub-band gap photoresponse measurements on the Si:Au photodiodes under 5 V reverse bias were performed with different sub-band gap wavelengths ( λ =1,310, 1,550 and 1,650 nm); spatially optimized external quantum efficiency (EQE) measurements for sub-band gap wavelengths for all Au doses are shown in Fig. 3f . Si:Au photodiode response increases monotonically with increasing gold concentration for all three sub-band gap wavelengths, with the maximum EQE of 2.8 × 10 −4 and 9.3 × 10 −5 for λ =1,310 and 1,550 nm, respectively. More detail about the EQE calculation can be found in the Methods section. Room-temperature spectral response of Si:Au photodiodes The extent and mechanism of Si:Au room-temperature optoelectronic spectral response was further studied via transient photoresponse measurements. Nanosecond pulses with tunable wavelengths ( λ =1,100–2,300 nm) were derived from an optical parametric amplifier (OPA) [44] pumped by a frequency-tripled, Q-switched Nd:YAG laser. The pulses were passed through a long pass filter and a Pellin Broca prism to eliminate any undesired wavelengths (for example, laser harmonics) before incidence n the photodiode. The shape of the spectral responses for the Si:Au photodiode with 1 × 10 15 cm −2 implant dose and the reference Si:B photodiode are shown in Fig. 4a . Because of the high intensity of the sub-band gap laser pulse, a sub-band gap photoresponse signal appeared within the reference silicon sample owing to two-photon absorption (TPA) [45] . This signal responded quadratically with pulse intensity, as expected for a two-photon process, and could be reduced by tuning the pulse intensity appropriately. The spectral response in the reference sample agrees well with the calculated value expected for TPA, I (λ) β (λ) where I (λ) is the intensity of the pulse laser used and β (λ) is the published value of two-photon absorption coefficient [45] for each wavelength (see Methods for the calculation of TPA). 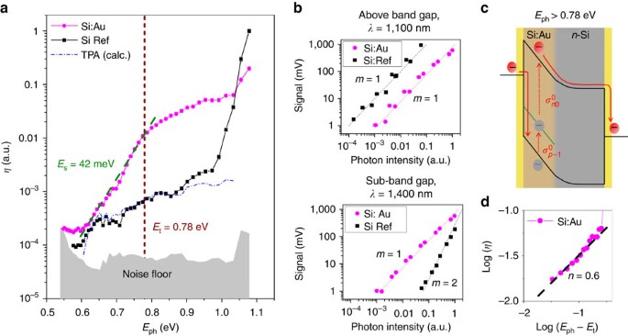Figure 4: Sub-band gap photoresponse mechanism of Si:Au. (a) Si:Au spectral responseηas a function of photon energy measured using tunable wavelength transient photoresponse measured at room temperature for the photodiode with the highest gold dose of 1015cm−2. A kink in the spectral response is observed at the threshold energyEt=0.78 eV, which corresponds to the substitutional gold donor level in silicon. ForEph<Et, the response is characterized by the Urbach absorption edge with a slope ofEs=42 meV. (b) Above-band gap and sub-band gap photoresponse of the Si:Au and reference silicon photodiodes for varying photon intensity, confirming that the sub-band gap response in the reference silicon is caused by two-photon absorption (TPA) in the substrate. Under standard operating conditions (~100 W cm−2or lower), no measurable TPA was observed in the reference silicon photodiode. (c) Possible sub-band gap photoresponse mechanism for substitutional gold in silicon through the donor level forEph>0.78 eV. (d) The polynomial dependence (n=0.6) ofηonEph, forEphclose toEt(0.8 eV<Eph<0.94 eV), suggesting that the defect-state wavefunction is close to that of a delta function. Figure 4: Sub-band gap photoresponse mechanism of Si:Au. ( a ) Si:Au spectral response η as a function of photon energy measured using tunable wavelength transient photoresponse measured at room temperature for the photodiode with the highest gold dose of 10 15 cm −2 . A kink in the spectral response is observed at the threshold energy E t =0.78 eV, which corresponds to the substitutional gold donor level in silicon. For E ph < E t , the response is characterized by the Urbach absorption edge with a slope of E s =42 meV. ( b ) Above-band gap and sub-band gap photoresponse of the Si:Au and reference silicon photodiodes for varying photon intensity, confirming that the sub-band gap response in the reference silicon is caused by two-photon absorption (TPA) in the substrate. Under standard operating conditions (~100 W cm −2 or lower), no measurable TPA was observed in the reference silicon photodiode. ( c ) Possible sub-band gap photoresponse mechanism for substitutional gold in silicon through the donor level for E ph >0.78 eV. ( d ) The polynomial dependence ( n =0.6) of η on E ph , for E ph close to E t (0.8 eV< E ph <0.94 eV), suggesting that the defect-state wavefunction is close to that of a delta function. Full size image Figure 4b shows the strength of the photoresponse signal with respect to the applied laser pulse intensity for both above gap and sub-band gap light. The photoresponse increased linearly with increasing laser pulse intensity except for the sub-band gap photoresponse in the reference silicon sample, which increased quadratically with increasing laser intensity due to TPA. In addition to the different scaling with photon intensity, the TPA signal was easily distinguished from the photoconductive signal because the transient decay of the response was much slower; this characteristic should be expected for TPA because free carriers were generated and had to be collected from the entire silicon substrate. To mitigate the effect of TPA from both Si:Au and reference silicon spectral response in Fig. 4a , only the short-lived peak of the transient signal was used in the definition of the dimensionless figure of merit η = A ·Δ I peak / N ph , where A =4.8 × 10 21 A −1 is a normalization constant, Δ I peak is the photo-generated current and N ph is the number of photons in the laser pulse. We observe measureable spectral response of Si:Au extending to E ph =0.55 eV, and a distinct change in slope at photon energy E ph =0.78 eV ( Fig. 4a ). This later spectral feature appears to be dopant specific, as discussed in the next section. We first comment on the probable origins of the sub-band gap photoresponse of Si:Au. Previous work by Sah et al . [46] and Okuyama et al . [48] utilized temperature-dependent photoconductivity and spectrally resolved low-temperature photoconductivity, respectively, to determine the energy level of gold impurities in silicon diffused with gold concentration below the solid solubility limit. At these low dopant concentrations, the Au-induced defect states are single, discrete levels with non-interacting localized states. In that study [48] , the reported spectral response has a distinct change in slope near the photon energy E ph =0.78 eV, which corresponds to the substitutional gold donor energy level in silicon. In our study, the same spectral feature was observed in the Si:Au photodiode with a gold dose of 1 × 10 15 cm −2 , suggesting that the sub-band gap photoresponse mechanism in these Si:Au photodiodes may be the same as that in gold-diffused silicon measured at liquid nitrogen temperature [48] . The higher gold concentration achieved by our PLM process apparently enables one to observe this effect at room-temperature. Next, we address the role of ‘drift’ in carrier extraction from the Si:Au layer. It is known that deep-level traps such as Au in silicon reduce the electronic carrier lifetime through non-radiative recombination [49] . With the gold concentration of N t =10 20 cm −3 and the saturated electron velocity of v s =10 7 cm s −1 assumed in the depleted Si:Au layer [50] , an electron trapping rate τ eo =( σ n t v s N t ) −1 =5 ps would be expected, given an electron capture cross-section σ n t =2 × 10 −16 cm 2 of gold in silicon [51] . Despite the low minority-carrier lifetime in Si:Au, some free electrons excited by the sub-band gap light in the hyperdoped region were able to escape into the n -type substrate. This process is aided because the Si:Au layer is fully depleted because of the low carrier concentration in gold-doped silicon (see Methods and Supplementary Fig. 3 ). This low carrier concentration in the Si:Au layer is believed to be caused by the self-compensation due to the ionization of deep acceptor and donor trap levels of substitutional gold in silicon [41] , [52] , [53] . The resulting full depletion of the Si:Au causes the majority of the applied reverse bias voltage to drop across this layer, thereby facilitating carrier transport via drift. This behaviour is in contrast with past work in sulphur-hyperdoped silicon [25] , where the free carrier concentration is between 10 17 and 10 20 cm –3 and the minority-carrier transport in the hyperdoped region is driven by the comparatively weaker process of diffusion [27] . The application of 5 V reverse bias across the hyperdoped layer appears sufficient to saturate the photoresponse. This is shown in Fig. 3c , where the photo-generated current produced by λ =1,550 nm light saturates with increasing reverse bias voltage. While higher gold concentration is expected to reduce the sub-band gap photoresponse by reducing the minority-carrier lifetime, the applied reverse bias voltage seems to be capable of overcoming the negative effect of higher gold concentration. Hence, the sub-band gap optoelectronic response increases with the increasing sub-band gap absorptance in samples with higher gold concentrations ( Fig. 3f ). Next, we discuss how the dopant type affects the infrared spectral response. In this dopant-mediated, extrinsic sub-band gap photoresponse mechanism, electrons can be excited into the conduction band through the dopant state(s). One probable mechanism is the electron excitation from the valence band to the conduction band through the donor energy level, which has previously been shown for gold-diffused silicon at low temperature ( Fig. 4c ) [48] , [54] . In ref. 28 , donor-assisted transition arises at threshold energy of 0.78 eV. Inspecting Fig. 4a , similar threshold energy is evident in the Si:Au photodiode. For photon energy E ph larger than the threshold energy E t =0.78 eV (ref. 34 ), the transitions characterized by photoionization cross-section (from valence band to the donor state) and (from donor state to the conduction band) are both possible. Electrons from the valence band can then be excited into the conduction band and swept away by the strong reverse bias electric field across the Si:Au layer into the n -type substrate. They are then transported as majority carriers in the conduction band before being extracted by the back contact. However, for E ph < E t the transition from the donor level to the conduction band characterized by is turned off; thus, electrons excited into the donor level eventually recombine into the valence band without leaving the Si:Au-hyperdoped region. As the donor-level/conduction-band transition is unavailable, the magnitude of the sub-band gap response for the energy range E ph < E t becomes exponentially less likely with decreasing excitation energy. One possible model for this exponential decay is the dependence η ( E ph ) exp(( E ph − E t )/ E s ) where E s is the slope of the Urbach absorption edge due to disorder in solids [55] . E s =42 meV has been extracted from fits to the experimental data as the slope of the Urbach edge. This is larger than kT =26 meV, suggesting that there is a disorder-induced broadening in either the impurity states or the conduction band edge of Si:Au. The spectral kink at E ph =0.78 eV closely matches the spectral response of gold-diffused silicon at low temperature, suggesting that it should be possible to tune the sub-band gap spectral response of hyperdoped silicon by using alternative dopant elements that introduce levels at different energies [48] . Further analysis can be done on the spectral response of Si:Au for E ph >0.78 eV. Various models have been proposed to explain the dependence of the photoionization cross-section σ ( E ph ) for deep levels in semiconductor. If the deep-level wavefunction is a localized state with delta function like spatial dependence in the length scale of the atomic radius, for E ph close to the threshold energy E t =0.78 eV the approximate dependence σ ( E ph ) ( E ph − E t ) 1/2 is expected [56] , [57] . In contrast, for a state with hydrogenic like wavefunction the approximate dependence σ ( E ph ) ( E ph − E t ) 3/2 is expected [58] . The conversion efficiency η is directly proportional to the photoionization cross-section in the Si:Au photodiode, and as such the dependence η ( E ph ) ( E ph − E t ) n for E ph close to E t =0.78 eV can be used to infer the spatial behaviour of the deep-level wavefunction. The range for the fit is set to 0.8 eV< E ph <0.94 eV to reduce the influence of the Urbach edge, and the fit is shown in Fig. 4d . The polynomial dependence of n =0.6 is extracted, suggesting that the deep-level state wavefunction for the donor level of Si:Au has a spatial dependence much closer to that of a delta function [56] , [57] than that of a hydrogenic wavefunction [58] . As the first demonstration devices, there is room to improve the absolute room-temperature sub-band gap EQE of ~10 −4 . Two focus areas should include improving sub-band gap light absorptance and incorporating best-in-class photodiode-design practices to enhance carrier collection. This can be achieved, for example, by using a larger gold implantation dose for the PLM process and applying an anti-reflection coating on the photodiode to increase the sub-band gap absorptance of the Si:Au layer beyond its current ~1% absorptance. Increasing the thickness of the Si:Au layer could also increase the optical path length and sub-band gap absorptance. Further gains may be possible via optimization of device design: because most of the gold dopants are concentrated near the silicon surface ( Fig. 1b ), the majority of free carriers generated by sub-band gap light are believed to be within the top 20 nm of the Si:Au surface. As the surface-limited lifetime for W =20 nm thick silicon is in the order of τ s = W / S =2 ps when a non-passivated surface recombination velocity S =10 6 cm s −1 is assumed [59] , the sub-band gap photoresponse in Si:Au with a bulk lifetime of ~5 ps is prone to surface recombination. Incorporating surface passivation could potentially suppress this recombination activity. We conservatively estimate that practical application of these improvements may increase the room temperature sub-band gap optoelectronic response of Si:Au photodiodes by two orders of magnitudes to EQE=10 −2 , although no physical limits are known at this time to prevent even higher EQE. In summary, we report the room-temperature sub-band gap optoelectronic response in silicon hyperdoped with gold using a two-step process: ion implantation followed by PLM. The sub-band gap optoelectronic response is shown to correspond to known gold dopant energy levels in silicon and increase with the implanted gold concentration. This work represents a fundamentally new approach to achieve sub-band gap optoelectronic response in silicon that avoids structural defects and interface management issues associated with combining foreign materials and silicon. While the magnitude of the room-temperature sub-band gap response demonstrated here is in the EQE~10 −4 range, further improvements are likely via device architecture optimization. The planar, single-crystal nature of the hyperdoped silicon layer created using the PLM process makes this an attractive material candidate for room-temperature sub-band gap photon-imaging devices based on silicon. Nanosecond PLM Silicon wafers (<100>, n -type, resistivity ~3 Ω cm, minority-carrier lifetime ~180 μs) were ion-implanted with 197 Au − at an energy of 50 keV, to doses of 3 × 10 14 , 7 × 10 14 or 1 × 10 15 atoms cm −2 . The wafers were then pulsed-laser melted by a single pulse from an Nd:YAG laser, using the third harmonic wavelength of 355 nm, with a pulse duration full-width-half-maximum (FWHM) of 5 ns and a fluence of 0.7 J cm −2 . The resulting material was characterized by SIMS using a Physical Electronics 6650 Dynamic SIMS instrument. Operating conditions were the following: 6 keV Cs ion beam at 1 nA, with SIMS craters being 50 μm 2 ; depth was measured ex situ by contact profilometry. Au concentrations were calibrated against known ion-implantation doses from the as-implanted regions of each sample, normalized by the [28] Si signal. Transmission electron microscopic samples were fabricated by focused-ion beam milling and liftout; transmission electron microscopic imaging was performed on a JEOL 2100 high-resolution transmission electron microscope operated at 200 keV in bright-field mode. Approximation of sub-band gap α in Si:Au We model the Si:Au as a uniform t =150 nm thin film on top of crystalline silicon wafer. It is assumed that the real refractive index of Si:Au is not any different from that of a normal crystalline silicon. Furthermore, to simplify the model, it is assumed that light interference in the thin-film Si:Au region does not play a critical role in the light propagation. As crystalline silicon does not absorb sub-band gap light, the sub-band gap light absorption in the Si:Au layer can then be approximated as: where A is the sub-band gap absorption measured using the spectrophotometer and R is the fraction of light reflected when light propagates through the air–silicon interface. Taking the value of R ~0.36 and A ~1%, α = A (1− R )/ t (1− R − AR )=600 cm −1 can be approximated. This is the lower bound for the value of α in Si:Au with gold implantation dose of 10 15 cm −2 . In reality, 90% of the gold atoms are buried within the top 20 nm of the Si:Au layer. As the majority of the sub-band gap light absorption is believed to occur within this 20 nm thin layer, the actual value of α in the region with highest gold concentration may be several times larger. Si:Au photodiode-type determination As we have detailed in the main text, at the supersaturated concentrations obtained for Si:Au implanted with gold doses of 3 × 10 14 , 7 × 10 14 and 1 × 10 15 cm −2 , the majority carriers in Si:Au are holes. When Si:Au is fabricated on an n -type silicon substrate, the resulting structure is a junction that shows the rectifying behaviour of a diode. In contrast, when Si:Au is fabricated on a p -type silicon substrate, the resulting structure does not rectify. A dark I–V curve for one such structure is shown in Supplementary Fig. 1 , where Si:Au with gold implantation dose of 10 14 cm −2 was fabricated on a p -type substrate. Photodiode device fabrication See Supplementary Fig. 2 for device dimensions. Before the PLM process, boron ions were selectively implanted into the gold-doped silicon area under the top contacts to improve contact resistance. The selected area for the boron implantation was patterned using photolithography, and [11] B + ions (3 × 10 14 cm −2 dose, 2 keV implantation energy) were implanted into the top 30 nm of the gold-doped area. The entire sample then underwent the PLM process (described above), creating a homogenous single-crystal Si:Au layer with a pair of rectangular Si:(Au+B)-patterned areas positioned for subsequent contact deposition. The depth of the boron doping is simulated to be ~70 nm deep after the PLM process. Photolithography and SF 6 reactive ion etch were then used to create a 1-μm-deep trench that isolated the 1 × 1 mm 2 rectangular Si:Au and the Si:(Au+B) contact area from the rest of the Si:Au layer. Photolithography, e -beam evaporation and lift-off were used to deposit 30/160 nm of Ti/Au contacts on top of the Si:(Au+B) areas. On the back of the silicon wafer, a uniform 30/160 nm Ti/Au layer was deposited across the entire surface as the photodiode back contact. The back contact was attached to an external electrode by conductive silver paste, while the top contacts were connected to electrodes by Al wire bonds. For the reference silicon photodiode, the same boron-doping profile is used everywhere instead of Si:Au, creating a p – n photodiode without any Au-hyperdoped silicon. EQE calculation A 2-V peak-to-peak square wave S ( t ) can be expressed as S ( t )=1.273 sin ( ωt )+0.4244, sin (3 ωt )+0.2546, sin ( ωt )+... where ω is the angular frequency and t is time. As the optically chopped light can be approximated as a square wave and the lock-in amplifier output V out is the root mean squared value of the first Fourier component of the signal, the mapped EQE for each coordinate on the photodiode can be calculated using the formula EQE( x , y )=2.22 V out ( x , y )/ Rqϕ ( λ ), where V out is the signal output from the lock-in amplifier, R is the value of the comparative resistor, q is the electron charge and ϕ ( λ ) is the number of photons incident on the sample per unit time measured using a calibrated germanium photodiode. The Si:Au photodiodes were operated at −5 V reverse bias for these EQE measurements. Modelling of fully depleted hyperdoped region in Si:Au diode When I–V responses of Si:Au photodiodes were measured under large reverse biases, it is observed that the dark current increases almost linearly with the increase of reverse bias voltage. This is in contrast to that of a non-depleted diode that normally approach a steady dark current following the diode equation I = I o ( e qV / kT −1). A simple diode model to simulate this behaviour is developed in the PC1D device simulator. A p -type emitter layer with a thickness of 150 nm and a low carrier lifetime of 20 ps is used to represent the Si:Au layer. The base is represented with an n -type silicon with 500 μm thickness and 180 μs carrier lifetime (parameter obtained from the actual substrate). PC1D simulation shows that the hyperdoped Si:Au region is indeed fully depleted, and that the resulting dark I–V curve shows the same linear behaviour for large reverse bias voltages ( Supplementary Fig. 3 ). Transient-pulse laser photoresponse The laser pulse with 10 ns FWHM exiting the OPA consisted of the sub-band gap signal wavelength ( λ s ), the idler wavelength ( λ i ), as well as possible leakage of other above-band gap wavelengths ( λ a ) due to the inner working of the OPA. λ a was first filtered out using a razor-edge 1,064 nm long pass edge filter (Edmund Optics, NT47-510). The resulting beam was further purified by dispersing it using Pellin Broca prism mounted on a rotation stage and selecting only the desired wavelength ( λ s ) with a subsequent aperture. The rotation stage was calibrated such that across the entire spectral range considered only λ s could illuminate the sample. Infrared neutral density filters mounted on a filter wheel were then used to tune the beam intensity. The intensity was chosen such that the magnitude of the transient voltage was much smaller than the supply voltage V in =−5 V to prevent signal saturation. Furthermore, the beam intensity was also chosen such that the signal due to two-photon absorption (TPA) in the substrate was minimized. An average of 200 pulses was used for the acquisition of each data point. TPA model for reference photodiode sub-band gap response One of the characteristics of two-photon absorption (TPA) is characterized by the sub-band gap absorption coefficient α TPA ( λ )= I ( λ ) β ( λ ) where I ( λ ) is the intensity of the pulse laser used and β ( λ ) is the published value of two-photon absorption coefficient [45] for each wavelength. The value of β ( λ ) for λ =1,200–2,200 nm is about 1 cm GW −1 . The maximum pulse laser energy in our transient photoresponse experiment is about 100 μJ per pulse with ~0.5 cm beam diameter. As the laser pulse FWHM is about 10 ns, the maximum instantaneous intensity of the laser pulses incident on the photodiode samples are 50 kW cm −2 . In this case, maximum α TPA ( λ ) of 5 × 10 −5 cm −1 can be approximated. This absorption coefficient is very small, and consequently for L =0.5 mm thick silicon reference photodiode that we used in our experiment the total sub-band gap light intensity absorbed due to TPA can be approximated as I ABS ( λ ) I ( λ )(1−exp(− α TPA ( λ )2 L )) I 2 ( λ ) β ( λ )2 L . The photoresponse signal observed in the oscilloscope is directly proportional to this value, hence the quadratic dependence of the signal to the photon intensity observed in Fig. 3b . The corresponding value for the dimensionless figure of merit η is obtained by dividing the photoresponse signal with the sub-band gap photon illumination. Hence, we have the proportionality relationship η ( λ )= AI ( λ ) β ( λ ) to model the two-photon absorption in Fig. 4a , where A is the normalization constant. How to cite this article: Mailoa, J. P. et al . Room-temperature sub-band gap optoelectronic response of hyperdoped silicon. Nat. Commun. 5:3011 doi: 10.1038/ncomms4011 (2014).